The gut microbiota suppresses insulin-mediated fat accumulation via the short-chain fatty acid receptor GPR43 The gut microbiota affects nutrient acquisition and energy regulation of the host, and can influence the development of obesity, insulin resistance, and diabetes. During feeding, gut microbes produce short-chain fatty acids, which are important energy sources for the host. Here we show that the short-chain fatty acid receptor GPR43 links the metabolic activity of the gut microbiota with host body energy homoeostasis. We demonstrate that GPR43-deficient mice are obese on a normal diet, whereas mice overexpressing GPR43 specifically in adipose tissue remain lean even when fed a high-fat diet. Raised under germ-free conditions or after treatment with antibiotics, both types of mice have a normal phenotype. We further show that short-chain fatty acid-mediated activation of GPR43 suppresses insulin signalling in adipocytes, which inhibits fat accumulation in adipose tissue and promotes the metabolism of unincorporated lipids and glucose in other tissues. These findings establish GPR43 as a sensor for excessive dietary energy, thereby controlling body energy utilization while maintaining metabolic homoeostasis. The gut microbiota is an assortment of microorganisms inhabiting the mammalian gastrointestinal tract, and recent research has demonstrated that the gut microbiota is involved in obesity and metabolic disorders [1] , [2] , [3] , [4] . Studies using high-fat diet (HFD)-induced obesity-related mice have linked an altered gut microbiota composition to the development of obesity, insulin resistance and diabetes in the host through several mechanisms, including increased energy harvest from the diet and altered fatty acid metabolism and composition in the adipose tissue and liver [5] , [6] , [7] , [8] . One important activity of the gut microbiota is to catabolize dietary fibres that are not completely hydrolysed by host enzymes [9] . The main colonic bacterial fermentation products of dietary fibre are short-chain fatty acids (SCFAs) such as acetate, propionate and butyrate [10] ; SCFAs can be utilized for de novo synthesis of lipids and glucose [11] , which are used as the main energy sources for the host. In addition to energy sources, SCFAs have been established as essential nutrients that also act as signalling molecules. Recently, two orphan G protein-coupled receptors, GPR41 and GPR43, have been reported to be activated by SCFAs [12] . GPR41 has been reported to couple to Gi/o as α-subunit of heterotrimeric G protein and act as a gut microbiota-related energy sensor in the sympathetic nervous system and the intestines [13] , [14] , [15] , [16] . GPR43 reportedly couples to either Gi/o or Gq as another α-subunit of heterotrimetric G protein [17] , [18] . GPR43 has also been reported to be expressed in the adipose tissue, intestines and immune tissues [19] , [20] . In the immune system, regulation of inflammatory responses by GPR43 is a well-studied process [20] , [21] , [22] ; however, GPR43 has not been as well studied in the adipose tissue. Some studies have indicated that GPR43 promotes leptin secretion, adipogenesis and inhibition of lipolysis in adipose tissue and adipocytes, thereby regulating energy metabolism [19] , [23] , [24] . HFD-fed GPR43-deficient mice exhibit improved glucose tolerance and reduced body fat mass [25] . On the other hand, other group reported that GPR43 expressed in the intestine improves glucose tolerance by promoting the secretion of glucagon-like peptide-1 (GLP-1; such as incretin) from L cells [26] . The roles of GPR43 in metabolic processes are still unclear. In this study, using mice lacking GPR43 and with adipose-specific overexpression of GPR43, we present the true function of GPR43 in the adipose tissue and the role of GPR43 in the regulation of the energy balance. Gpr43 is abundantly expressed in the white adipose tissue Gpr43 was mainly expressed in the immune tissue and the white adipose tissue (WAT) of adult mice, as previously reported [18] , [19] , but not in the brown adipose tissue (BAT; Fig. 1a ). In situ hybridization at the postnatal stage (P1) confirmed that Gpr43 was most abundantly expressed in the WAT and was not expressed in the BAT ( Fig. 1b ). During adipogenesis, Gpr43 was expressed in the later stages of differentiation than aP2 and PPARg , markers of mature adipocytes (MAs) in 3T3-L1 pre-adipocytes and mouse embryonic fibroblasts (MEFs; Fig. 1c ). In the adult mouse adipose tissue, Gpr43 was abundantly expressed in the MA fraction but not in the stromal vascular fraction, containing pre-adipocytes and macrophages ( Fig. 1d ). Moreover, Gpr43 expression was markedly higher in the WAT of HFD-fed mice as compared with normal chow (NC)-fed mice ( Fig. 1e ). Thus, Gpr43 was abundantly expressed in the mature WAT but not in the BAT or in pre-adipocytes. 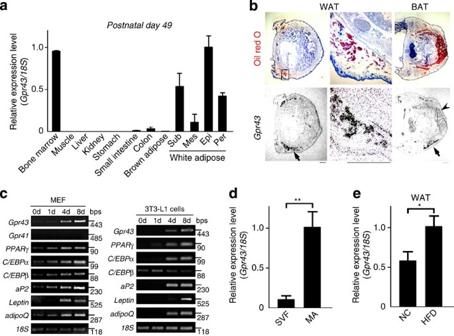Figure 1:Gpr43is abundantly expressed in the WATs. (a)Gpr43expression in postnatal mouse tissues (P49) measured by qRT-PCR (n=3). Internal control:18SrRNA expression. (b)Gpr43mRNA localization in mouse embryos (P1) as determined byin situhybridization using an35S-labelled antisenseGpr43RNA probe. Black grains superimposed on haematoxylin−eosin (H&E) and oil red O-stained sections indicateGpr43mRNA localization. Arrow indicates WAT; arrowhead indicates BAT. Scale bar, 1 mm. (c) Expression ofGpr43mRNA during differentiation. MEF and 3T3-L1 pre-adipocytes were induced to differentiate in the presence of MDI. Total RNA was analysed by RT-PCR.18Swas used as a loading control. (d)Gpr43expression in stromal vascular fraction (SVF) and MAs measured by qRT-PCR (n=3).18Swas used as a loading control. (e)Gpr43expression in the WAT of NC and HFD-fed mice measured by qRT-PCR (n=4);18Swas used as a loading control. Mice were analysed at 16 weeks of age (d,e). All data are presented as mean±s.e.m. Student’st-test; *P<0.05; **P<0.005. Epi, epididymal; Mes, mesenteric; Per, perirenal; Sub, subcutaneous. Figure 1: Gpr43 is abundantly expressed in the WATs. ( a ) Gpr43 expression in postnatal mouse tissues (P49) measured by qRT-PCR ( n =3). Internal control: 18S rRNA expression. ( b ) Gpr43 mRNA localization in mouse embryos (P1) as determined by in situ hybridization using an 35 S-labelled antisense Gpr43 RNA probe. Black grains superimposed on haematoxylin−eosin (H&E) and oil red O-stained sections indicate Gpr43 mRNA localization. Arrow indicates WAT; arrowhead indicates BAT. Scale bar, 1 mm. ( c ) Expression of Gpr43 mRNA during differentiation. MEF and 3T3-L1 pre-adipocytes were induced to differentiate in the presence of MDI. Total RNA was analysed by RT-PCR. 18S was used as a loading control. ( d ) Gpr43 expression in stromal vascular fraction (SVF) and MAs measured by qRT-PCR ( n =3). 18S was used as a loading control. ( e ) Gpr43 expression in the WAT of NC and HFD-fed mice measured by qRT-PCR ( n =4); 18S was used as a loading control. Mice were analysed at 16 weeks of age ( d , e ). All data are presented as mean±s.e.m. Student’s t -test; * P <0.05; ** P <0.005. Epi, epididymal; Mes, mesenteric; Per, perirenal; Sub, subcutaneous. Full size image Gpr43 knockout mice exhibit obesity To clarify the function of GPR43 in the WAT, we generated Gpr43−/− mice ( Supplementary Fig. S1a–d ). The Gpr43−/− mice showed no difference in the WAT area compared with wild-type mice at the embryonic stage (P1; Fig. 2a ), indicating that GPR43 had no effect on adipocyte differentiation. However, the body weights and WAT weights of both NC- and HFD-fed Gpr43−/− mice were significantly higher than that of wild-type mice during growth ( Fig. 2b ). Differences in the body weight between wild-type and Gpr43−/− mice were enhanced in an HFD-fed condition. The food intake was comparable between wild-type and Gpr43−/− mice fed an NC but was higher in Gpr43−/− mice fed an HFD ( Supplementary Fig. S2a ). In contrast, the plasma leptin levels were similar between wild-type and Gpr43−/− mice fed an HFD ( Supplementary Fig. S2b ). A significant increase in adipocyte size in WAT ( Fig. 2d ), but not BAT ( Supplementary Fig. S2c ), was also observed in HFD-fed Gpr43−/− mice. Furthermore, messenger RNA and protein expression of aP2 and PPARg were enhanced in the WAT of HFD-fed Gpr43−/− mice ( Fig. 2e ), while mRNA expression of PPARg and UCP1 , a thermogenesis marker, in the BAT was not significantly changed ( Supplementary Fig. S2d ). Moreover, HFD-induced insulin resistance, as determined by insulin tolerance test (ITT) and glucose tolerance test (GTT), was significantly increased in Gpr43−/− mice, compared with wild-type mice, whereas they were no differences in NC-fed mice ( Fig. 2g ). During insulin clamp studies, the glucose infusion rate (GIR) required to maintain euglycaemia, glucose rate of disappearance (Rd) and suppression of hepatic glucose production (HGP) were significantly decreased in HFD-fed Gpr43−/− mice compared with HFD-fed wild-type mice ( Fig. 2i ). Thus, these results indicate the decreased insulin sensitivity in HFD-fed Gpr43−/− mice. Furthermore, HFD-fed Gpr43−/− mice exhibited an increase in F4/80-positive macrophages, compared with HFD-fed wild-type mice ( Fig. 2j , left panel). The expression of F4/80 ( Fig. 2j , middle panel) and the inflammatory marker gene TNFa ( tumour necrosis factor α ) ( Fig. 2j , right panel) in both NC- and HFD-fed Gpr43−/− mice markedly increased, compared with wild-type mice. Thus, Gpr43−/− mice showed progression of inflammation accompanying the obese phenotype. 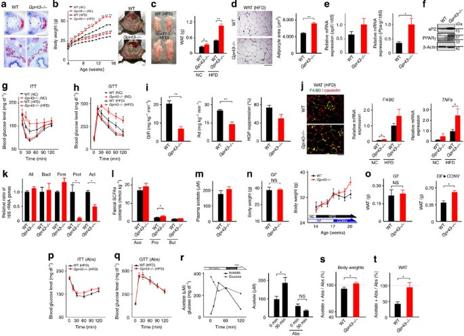Figure 2:Gpr43knockout mice are obese. (a) WAT and BAT of littermates (P1) were stained with oil red O. Scale bar: 5 mm (upper), 100 μm (lower). Body weight (b,n=10, 11) and fat mass (c,n=6–10) changes. Scale bar, 1 cm. (d) Haematoxylin–eosin (H&E)-stained WAT and mean area of adipocytes (n=3). Scale bar, 100 μm. Expression ofaP2andPpargmRNA (e,n=4) and protein (f) in the WAT of HFD-fed mice. ITT (g,n=4–6) and GTT (h,n=6, 7). (i) Euglycaemic hyperinsulinaemic clamp in HFD-fed mice. Left: glucose infusion ratio; middle: glucose disposal rate; right: hepatic glucose production suppression. Body weights; WT (33±2.9 g):Gpr43−/−(39±1.7 g), 14–15 weeks of age (n=4). (j) Level of inflammation (left panel) and expression ofF4/80(middle panel,n=4, 5) andTNFa(right panel,n=4−6) mRNA in WAT. Scale bar, 100 μm. (k) Comparison of microbial communities in HFD-fed mice, as assessed by qPCR (n=4). Act, actinobacteria; All, all bacteria; Bact, bacteroidetes; Firm, firmicutes; Prot, γ-proteobacteria. (l,m) Faecal major SCFA and plasma acetate contents in HFD-fed mice (n=4). Ace, acetate; But, butyrate; Pro, propionate. (n) Body weights of HFD-fed mice under GF conditions (20 weeks) (n=4, 6) (left panel). Body weight changes under GF to CONV conditions (n=4–6) (right panel). (o) Fat mass in 18-week-old mice under GF condition (n=4, 6) and 22-week-old mice on HFD under CONV conditions after 16 weeks of GF conditions (n=4, 5). (p,q) ITT and GTT under antibiotic treatment (n=4). Abs, antibiotics. (r) Acetate and glucose plasma concentrations after 1 h of feeding (24 h fasting) (left panel). Plasma acetate concentration with or without antibiotic treatment during feeding (right panel) (n=4). (s,t) Effect of acetate on body weights and fat mass under antibiotic treatment (n=6). Mice were analysed at 14 or 16 weeks of age. All data are presented as mean±s.e.m. Student’st-test; *P<0.05; **P<0.005; NS, not significant. Figure 2: Gpr43 knockout mice are obese. ( a ) WAT and BAT of littermates (P1) were stained with oil red O. Scale bar: 5 mm (upper), 100 μm (lower). Body weight ( b , n =10, 11) and fat mass ( c , n =6–10) changes. Scale bar, 1 cm. ( d ) Haematoxylin–eosin (H&E)-stained WAT and mean area of adipocytes ( n =3). Scale bar, 100 μm. Expression of aP2 and Pparg mRNA ( e , n =4) and protein ( f ) in the WAT of HFD-fed mice. ITT ( g , n =4–6) and GTT ( h , n =6, 7). ( i ) Euglycaemic hyperinsulinaemic clamp in HFD-fed mice. Left: glucose infusion ratio; middle: glucose disposal rate; right: hepatic glucose production suppression. Body weights; WT (33±2.9 g): Gpr43−/− (39±1.7 g), 14–15 weeks of age ( n =4). ( j ) Level of inflammation (left panel) and expression of F4/80 (middle panel, n =4, 5) and TNFa (right panel, n =4−6) mRNA in WAT. Scale bar, 100 μm. ( k ) Comparison of microbial communities in HFD-fed mice, as assessed by qPCR ( n =4). Act, actinobacteria; All, all bacteria; Bact, bacteroidetes; Firm, firmicutes; Prot, γ-proteobacteria. ( l , m ) Faecal major SCFA and plasma acetate contents in HFD-fed mice ( n =4). Ace, acetate; But, butyrate; Pro, propionate. ( n ) Body weights of HFD-fed mice under GF conditions (20 weeks) ( n =4, 6) (left panel). Body weight changes under GF to CONV conditions ( n =4–6) (right panel). ( o ) Fat mass in 18-week-old mice under GF condition ( n =4, 6) and 22-week-old mice on HFD under CONV conditions after 16 weeks of GF conditions ( n =4, 5). ( p , q ) ITT and GTT under antibiotic treatment ( n =4). Abs, antibiotics. ( r ) Acetate and glucose plasma concentrations after 1 h of feeding (24 h fasting) (left panel). Plasma acetate concentration with or without antibiotic treatment during feeding (right panel) ( n =4). ( s , t ) Effect of acetate on body weights and fat mass under antibiotic treatment ( n =6). Mice were analysed at 14 or 16 weeks of age. All data are presented as mean±s.e.m. Student’s t -test; * P <0.05; ** P <0.005; NS, not significant. Full size image We next examined the effects of the gut microbiota in the WAT. Communities of gut microbiota in Gpr43−/− mice exhibited an increase in Firmicutes, an SCFA-producing phylum, and a decrease in γ-proteobacteria and actinobacteria ( Fig. 2k ). Faecal SCFA and plasma acetate concentrations in Gpr43−/− mice increased compared with wild-type mice ( Fig. 2l ). Treatment with antibiotics lowered the total gut microbiota load by 90% and caused enlargement of the ceca ( Supplementary Fig. S2e ), similar to observation in germ-free (GF) mice [27] , then faecal SCFAs were markedly decreased ( Supplementary Fig. S2f ). Plasma acetate decreased significantly by antibiotic treatment and under GF conditions, which was recovered by returning to conventional (CONV) conditions ( Supplementary Fig. S2g ). Interestingly, differences in the body weights and WAT weights between HFD-fed Gpr43−/− and wild-type mice were completely abolished under GF conditions ( Fig. 2n (left panel) and 2o ). The difference could be observed again after returning to CONV conditions ( Fig. 2n (right panel) and 2o ). Moreover, under antibiotic treatment, the difference in insulin resistance of wild-type and Gpr43−/− mice by ITT and GTT was abolished ( Fig. 2p ). During feeding, the acetate level was increased after the rise in glucose, which was completely abolished by treatment with antibiotics ( Fig. 2r ). We found that administration of acetate during antibiotic treatment recovered the plasma acetate levels to that under normal conditions ( Supplementary Fig. S2g ). In addition, the body weight and WAT weight decreased significantly by administration of acetate with antibiotic treatment in wild-type mice, whereas these effects were not exhibited in Gpr43−/− mice ( Fig. 2s ). These results suggested that the GPR43 function is closely linked with the SCFAs produced by the gut microbiota. Adipose-specific Gpr43 transgenic mice are lean To determine whether the obesity in Gpr43−/− mice was due to the deficiency of GPR43 in the adipose tissue and not in the immune system and the intestines, we generated aP2 promoter-driven adipose-specific Gpr43 transgenic mice ( aP2-Gpr43TG ; Supplementary Fig. S1e–h ). Similar to Gpr43−/− mice, aP2-Gpr43TG mice also showed no difference in the WAT area during adipogenesis, as compared with wild-type mice at the embryonic stage (P1; Fig. 3a ). On the other hand, the body weights and WAT weights of aP2-Gpr43TG mice were significantly lower than those of wild-type mice during growth ( Fig. 3b ). However, while the food intake was comparable ( Supplementary Fig. S2h ), the plasma leptin level was significantly reduced in aP2-Gpr43TG mice compared with wild-type mice ( Supplementary Fig. S2i ). The adipocyte size in the WAT of aP2-Gpr43TG mice was significantly smaller than that of wild-type mice ( Fig. 3d ). Furthermore, the mRNA and protein expression of aP2 and PPARg decreased in the WAT of aP2-Gpr43TG mice ( Fig. 3e ). Compared with the alterations observed in Gpr43−/− mice, communities of gut microbiota were not dramatically different between wild-type and aP2-Gpr43TG ( Fig. 3g ); however, faecal SCFA and plasma acetate concentrations in aP2-Gpr43TG mice were higher compared with those in wild-type mice ( Fig. 3h ). These data indicate that the alteration of gut microbiota communities observed in Gpr43−/− mice is not dependent on the function of GPR43 expressed in adipose tissues; however, GPR43 in other tissues, such as the immune system, maybe involved in this alteration. Differences in the body weight and WAT weight between wild-type and aP2-Gpr43TG mice were also completely abolished by antibiotic treatment ( Fig. 3j ). 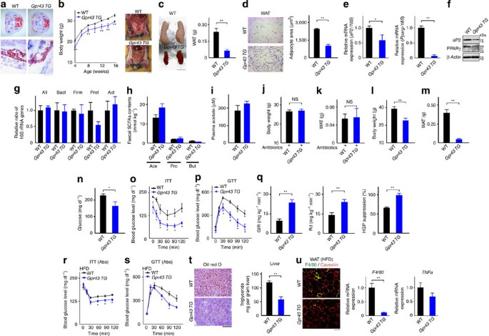Figure 3: Adipose tissue-specificGpr43transgenic mice are lean. (a) Subcutaneous WAT and interscapular BAT of littermates (P1) were stained with oil red O. Scale bar: 5 mm (upper), 100 μm (lower). Body weight changes (b,n=6–8) and fat mass (c,n=6, 5). Scale bar, 1 cm. (d) Haematoxylin–eosin (H&E)-stained epididymal WAT and mean area of adipocytes (n=4, 3). Scale bar, 100 μm. Expression ofaP2andPpargmRNA (e,n=6, 5) and protein (f) in the WAT; β-actin was used as a loading control. (g) Comparison of microbial communities, as assessed by qPCR (n=4). Faecal major SCFA (h,n=4) and plasma acetate (i,n=5) contents inaP2-Gpr43TGmice fed an HFD (n=4). Body weight (j) and fat mass (k) under antibiotic treatment (n=7, 6). Body weight (l) and fat mass (m) ofaP2-Gpr43TGmice fed an HFD (n=7). (n) Plasma glucose concentration inaP2-Gpr43TGmice fed an HFD (n=6). ITT (o) and GTT (p) inaP2-Gpr43 TGmice fed an HFD (n=6, 5). (q) Euglycaemic hyperinsulinaemic clamp in aP2-Gpr43TGmice fed an HFD. Left: glucose infusion ratio; middle: glucose disposal rate; right: hepatic glucose production suppression. Body weights; WT (44±1.3 g):aP2-Gpr43TG(33±1.1 g), 17 weeks of age (n=6, 5). ITT (r) and GTT (s) inaP2-Gpr43TGmice fed an HFD under antibiotic treatment (n=3). (t) Oil red O-stained liver and hepatic triglyceride content inaP2-Gpr43 TGmice fed an HFD (n=6, 4). Scale bar, 100 μm. (u) Level of WAT inflammation. Merged images from WAT, costained with anti-F4/80 (green) and anti-caveolin1 (red) antibodies (left panel). Scale bar, 100 μm. Expression ofF4/80(middle panel,n=4–5) andTNFa(right panel,n=4–6) mRNA in the WAT. Mice were analysed at 16 weeks of age. All data are presented as mean±s.e.m. Student’st-test; *P<0.05; **P<0.005; NS, not significant. Figure 3: Adipose tissue-specific Gpr43 transgenic mice are lean. ( a ) Subcutaneous WAT and interscapular BAT of littermates (P1) were stained with oil red O. Scale bar: 5 mm (upper), 100 μm (lower). Body weight changes ( b , n =6–8) and fat mass ( c , n =6, 5). Scale bar, 1 cm. ( d ) Haematoxylin–eosin (H&E)-stained epididymal WAT and mean area of adipocytes ( n =4, 3). Scale bar, 100 μm. Expression of aP2 and Pparg mRNA ( e , n =6, 5) and protein ( f ) in the WAT; β-actin was used as a loading control. ( g ) Comparison of microbial communities, as assessed by qPCR ( n =4). Faecal major SCFA ( h , n =4) and plasma acetate ( i , n =5) contents in aP2-Gpr43TG mice fed an HFD ( n =4). Body weight ( j ) and fat mass ( k ) under antibiotic treatment ( n =7, 6). Body weight ( l ) and fat mass ( m ) of aP2-Gpr43TG mice fed an HFD ( n =7). ( n ) Plasma glucose concentration in aP2-Gpr43TG mice fed an HFD ( n =6). ITT ( o ) and GTT ( p ) in aP2-Gpr43 TG mice fed an HFD ( n =6, 5). ( q ) Euglycaemic hyperinsulinaemic clamp in aP2- Gpr43TG mice fed an HFD. Left: glucose infusion ratio; middle: glucose disposal rate; right: hepatic glucose production suppression. Body weights; WT (44±1.3 g): aP2-Gpr43TG (33±1.1 g), 17 weeks of age ( n =6, 5). ITT ( r ) and GTT ( s ) in aP2-Gpr43TG mice fed an HFD under antibiotic treatment ( n =3). ( t ) Oil red O-stained liver and hepatic triglyceride content in aP2-Gpr43 TG mice fed an HFD ( n =6, 4). Scale bar, 100 μm. ( u ) Level of WAT inflammation. Merged images from WAT, costained with anti-F4/80 (green) and anti-caveolin1 (red) antibodies (left panel). Scale bar, 100 μm. Expression of F4/80 (middle panel, n =4–5) and TNFa (right panel, n =4–6) mRNA in the WAT. Mice were analysed at 16 weeks of age. All data are presented as mean±s.e.m. Student’s t -test; * P <0.05; ** P <0.005; NS, not significant. Full size image Next, we examined the effects of overexpressing GPR43 in the WAT on HFD-induced obesity. Increases in the body weight, WAT weight and blood glucose by HFD-induced obesity were markedly suppressed in aP2-Gpr43TG mice ( Fig. 3l–n ). Moreover, HFD-induced insulin resistance, as determined by ITT and GTT, was significantly attenuated in aP2-Gpr43TG ( Fig. 3o ). During insulin clamp studies, in contrast to Gpr43−/− mice, the GIR, Rd and HGP suppression in HFD-fed aP2-Gpr43TG mice were significantly increased, compared with HFD-fed wild-type mice ( Fig. 3q ). Moreover, under antibiotic treatment, the difference in insulin resistance of wild-type and aP2-Gpr43TG mice was attenuated ( Fig. 3r ). HFD-induced obesity caused liver steatosis and high hepatic triglyceride content in wild-type mice but not in aP2-Gpr43TG mice ( Fig. 3t ). Furthermore, HFD-fed aP2 - Gpr43TG mice exhibited a decrease in F4/80-positive macrophages, compared with HFD-fed wild-type mice ( Fig. 3u , left panel) and the expression of F4/80 ( Fig. 3u , middle panel) and TNFa ( Fig. 3u , right panel) in aP2-Gpr43TG mice was decreased. On the basis of the data for aP2-Gpr43TG mice, we concluded that progression of inflammation in KO mice was mainly caused by obesity; however, we do not exclude the possibility that deletion of GPR43 in the immune system enhances inflammation in WAT. These results showed that overexpressing GPR43 suppressed HFD-induced obesity and improved insulin sensitivity. GPR43 suppresses insulin signalling in adipose tissue We further examined the relationship between GPR43 function and insulin sensitivity. The WAT, muscles and liver are the three major tissues involved in fuel metabolism [28] . Surprisingly, although insulin sensitivity was improved in aP2-Gpr43TG mice compared with wild-type mice in the context of HFD feeding ( Fig. 3o ), insulin-induced Akt phosphorylation in the WAT, but not the muscles or liver, was markedly suppressed ( Fig. 4a–c ). Administration of acetate significantly suppressed insulin-induced Akt phosphorylation in the WAT, but not the muscles or liver of wild-type mice, whereas the effect was not exhibited in the WAT of Gpr43−/− mice ( Fig. 4d–f ). These results indicated that GPR43 signalling suppressed insulin signalling only in the WAT. 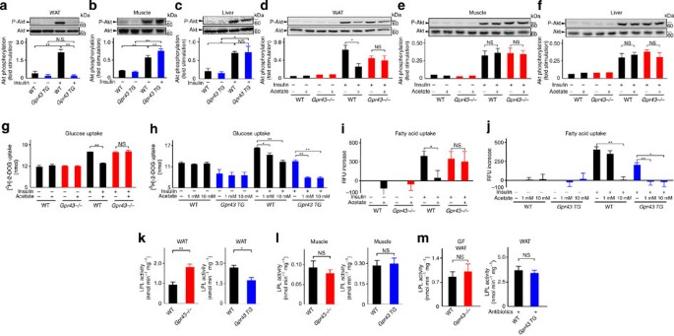Figure 4: GPR43 suppresses insulin signalling in the adipose tissues but not in muscles or liver. Insulin-stimulated Akt phosphorylation of Ser473 in the WAT (a,n=3), muscles (b,n=4) and liver (c,n=3) ofaP2-Gpr43TGmice fed an HFD after 6 h of fasting. (d–f) Inhibitory effects of acetate on insulin signalling (1 g kg−1, i.p.). After pretreatment with acetate for 40 min, a bolus of insulin (0.15 U kg−1) with or without acetate (1 g kg−1) was administered intraperitoneally. Akt phosphorylation of Ser473 in the WAT (d,n=3), muscles (e,n=3) and liver (f,n=3) ofGpr43−/− mice after 6 h of fasting. (g,h) Effect of acetate on glucose uptake in MEF-derived adipocytes fromGpr43−/−oraP2-Gpr43TGmice (n=4, respectively). (i,j) Effect of acetate on the fatty acid uptake in MEF-derived adipocytes fromGpr43−/−oraP2-Gpr43TGmice (n=8–15). LPL activity in the WAT (k,n=4–5) and the muscles (l,n=3–5) ofGpr43−/−oraP2-Gpr43TGmice (n=3–4). (m) LPL activity ofGpr43−/−mice fed an HFD under GF conditions (n=4, 6) oraP2-Gpr43TGmice treated with antibiotics (n=7, 6). All mice were analysed at 15–16 weeks of age. All data are presented as mean±s.e.m. analysis of variance followed by Tukey–Kramer’spost hoctest (a–j) and Student’st-test (k–m); *P<0.05; **P<0.005; NS, not significant. Figure 4: GPR43 suppresses insulin signalling in the adipose tissues but not in muscles or liver. Insulin-stimulated Akt phosphorylation of Ser473 in the WAT ( a , n =3), muscles ( b , n =4) and liver ( c , n =3) of aP2-Gpr43TG mice fed an HFD after 6 h of fasting. ( d – f ) Inhibitory effects of acetate on insulin signalling (1 g kg −1 , i.p.). After pretreatment with acetate for 40 min, a bolus of insulin (0.15 U kg −1 ) with or without acetate (1 g kg −1 ) was administered intraperitoneally. Akt phosphorylation of Ser473 in the WAT ( d , n =3), muscles ( e , n =3) and liver ( f , n =3) of Gpr43 −/− mice after 6 h of fasting. ( g , h ) Effect of acetate on glucose uptake in MEF-derived adipocytes from Gpr43−/− or aP2-Gpr43TG mice ( n =4, respectively). ( i , j ) Effect of acetate on the fatty acid uptake in MEF-derived adipocytes from Gpr43−/− or aP2-Gpr43TG mice ( n =8–15). LPL activity in the WAT ( k , n =4–5) and the muscles ( l , n =3–5) of Gpr43−/− or aP2-Gpr43TG mice ( n =3–4). ( m ) LPL activity of Gpr43−/− mice fed an HFD under GF conditions ( n =4, 6) or aP2-Gpr43TG mice treated with antibiotics ( n =7, 6). All mice were analysed at 15–16 weeks of age. All data are presented as mean±s.e.m. analysis of variance followed by Tukey–Kramer’s post hoc test ( a – j ) and Student’s t -test ( k – m ); * P <0.05; ** P <0.005; NS, not significant. Full size image Hence, we next examined the functions of SCFAs and GPR43 on WAT insulin signalling-related bioactivity [29] . GPR43 promotes adipogenesis in vitro [19] . Thus, to avoid variations in the differentiation of adipocytes by GPR43 deficiency, we used pioglitazone-induced adipogenesis [30] . As expected, adipogenesis in pioglitazone-enhanced MEF-derived adipocytes did not differ in wild-type and Gpr43−/− or aP2-GPR43TG mice ( Supplementary Fig. S3a,b ). Acetate significantly suppressed the insulin-induced glucose and fatty acid uptake in adipocytes from wild-type mice but not Gpr43−/− mice ( Fig. 4g ; Supplementary Fig. S3c ), whereas it was further enhanced in adipocytes from aP2-Gpr43TG mice ( Fig. 4h ). Moreover, the lipoprotein lipase (LPL) activity was higher in HFD-fed Gpr43−/− mice, and lower in aP2-Gpr43TG in the WAT but not in muscle ( Fig. 4k ). These effects on the LPL activity in the WAT were abolished under GF conditions and by antibiotic treatment ( Fig. 4m ). In addition, Lpl mRNA expression in the WAT was comparable in Gpr43−/− mice, and lower in aP2-Gpr43TG mice ( Supplementary Fig. S3d ). Collectively, these results indicated that suppression of insulin signalling in the WAT, but not the muscles or liver, altered the glucose and lipid metabolism by acetate-dependent GPR43 stimulation. GPR43 suppresses insulin signalling via G(i/o)βγ–PLC–PKC–PTEN We further examined the GPR43-mediated intracellular signalling in 3T3-L1 pre-adipocyte-derived adipocytes. Phenylacetamide (PA) is known as a GPR43-selective agonist [31] , while cyclopropanecarboxylic acid is a partially selective GPR41 agonist ( Supplementary Fig. S4a,b ). Acetate and PA significantly suppressed insulin-induced Akt phosphorylation, whereas cyclopropanecarboxylic acid weakly suppressed the same ( Fig. 5a ). On the other hand, N 6 -cyclopentyladenosine, a ligand for the adenosine A1 receptor (Gi/o-type G protein-coupled receptor) [32] had no effects on insulin-induced Akt phosphorylation ( Supplementary Fig. S4c ). GPR43-mediated suppression of insulin-induced Akt phosphorylation was effectively blocked by the treatment with pertussis toxin (PTX), a Gi/o-type G protein inactivator [33] ( Fig. 5b ), whereas the treatment of short interfering RNA (siRNA) against Gq protein ( Supplementary Fig. S4d,e ) had no inhibitory effects ( Fig. 5c ). Moreover, GPR43-mediated suppression of insulin-induced Akt phosphorylation was effectively blocked by the treatment with Gallein (Gβγ blocker) but not NF023 (Gα(i/o) blocker [14] ) ( Fig. 5b ). It is reported that G(i/o)βγ mediates to the PLC–PKC–ERK pathway [34] . GPR43-mediated suppression of insulin-induced Akt phosphorylation was effectively blocked by the treatment with U73122 (PLC inhibitor) and Go6983 (PKC inhibitor), but not U0126 (MEK inhibitor) ( Fig. 5d ). 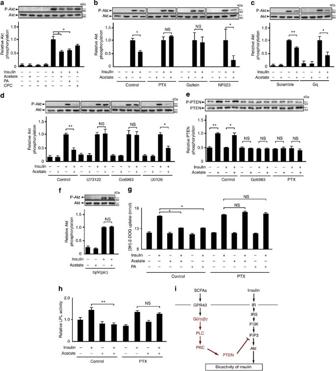Figure 5: GPR43 suppresses insulin signalling via G(i/o)βγ-PLC–PKC–PTEN signalling. (a) Inhibitory effects of GPR43 agonists (10 mM acetate and 10 μM PA) and a GPR41 agonist (10 μM cyclopropanecarboxylic acid (CPC)) on insulin-induced Akt phosphorylation (n=3). PA, phenylacetamide. (b) Effects of Gi/o signalling inhibition on suppression of insulin-induced Akt phosphorylation by acetate (n=3). (c) Effects of Gq signalling inhibition using siRNA (no. 1) on suppression of insulin-induced Akt phosphorylation by acetate (n=3). (d) Effects of Gβγ signalling inhibition on suppression of insulin-induced Akt phosphorylation by acetate (n=3). (e) Effects of GPR43 stimulation on PTEN phosphorylation (n=3). (f) Effects of PTEN signalling inhibition on suppression of insulin-induced Akt phosphorylation by acetate (n=3). Cells were stimulated with insulin (3 μg ml−1) in the presence of acetate (10 mM) and bpV(pic) (1 μM) for 5 min after pretreatment with acetate for 2 h. (g) Effect of GPR43 agonists (10 mM acetate and 10 μM PA) on insulin-induced glucose uptake (n=4). (h) Effect of acetate on insulin-induced LPL activity (n=4). Cells were stimulated with insulin (3 μg ml−1) in the presence of acetate (10 mM) and inhibitor for 30 min after pretreatment with acetate for 2 h and PTX (1 μg ml−1) for 4 h. In all experiments, cells were stimulated with insulin (3 μg ml−1) in the presence of GPR43 agonist (10 mM acetate, 10 μM PA, or 10 μM CPC) for 5 min after pretreatment with GPR43 agonists for 2 h, Gallein (10 μM), NF023 (10 μM), PTX (1 μg ml−1), U73122 (1 μM), Go6983 (10 μM),or U0126 (10 μM) for 4 h. All experiments were performed by using 3T3-L1-derived adipocytes (a–f,h) and MEF-derived adipocytes (g). All data are presented as mean±s.e.m. analysis of variance followed by Tukey–Kramer’spost hoctest; *P<0.05; **P<0.005; NS, not significant. (i) Schematic diagram of the mechanism for GPR43-mediated suppression of fat accumulation. Novel GPR43 signalling events in adipocytes are shown in red. Figure 5: GPR43 suppresses insulin signalling via G(i/o)βγ-PLC–PKC–PTEN signalling. ( a ) Inhibitory effects of GPR43 agonists (10 mM acetate and 10 μM PA) and a GPR41 agonist (10 μM cyclopropanecarboxylic acid (CPC)) on insulin-induced Akt phosphorylation ( n =3). PA, phenylacetamide. ( b ) Effects of Gi/o signalling inhibition on suppression of insulin-induced Akt phosphorylation by acetate ( n =3). ( c ) Effects of Gq signalling inhibition using siRNA (no. 1) on suppression of insulin-induced Akt phosphorylation by acetate ( n =3). ( d ) Effects of Gβγ signalling inhibition on suppression of insulin-induced Akt phosphorylation by acetate ( n =3). ( e ) Effects of GPR43 stimulation on PTEN phosphorylation ( n =3). ( f ) Effects of PTEN signalling inhibition on suppression of insulin-induced Akt phosphorylation by acetate ( n =3). Cells were stimulated with insulin (3 μg ml −1 ) in the presence of acetate (10 mM) and bpV(pic) (1 μM) for 5 min after pretreatment with acetate for 2 h. ( g ) Effect of GPR43 agonists (10 mM acetate and 10 μM PA) on insulin-induced glucose uptake ( n =4). ( h ) Effect of acetate on insulin-induced LPL activity ( n =4). Cells were stimulated with insulin (3 μg ml −1 ) in the presence of acetate (10 mM) and inhibitor for 30 min after pretreatment with acetate for 2 h and PTX (1 μg ml −1 ) for 4 h. In all experiments, cells were stimulated with insulin (3 μg ml −1 ) in the presence of GPR43 agonist (10 mM acetate, 10 μM PA, or 10 μM CPC) for 5 min after pretreatment with GPR43 agonists for 2 h, Gallein (10 μM), NF023 (10 μM), PTX (1 μg ml −1 ), U73122 (1 μM), Go6983 (10 μM),or U0126 (10 μM) for 4 h. All experiments were performed by using 3T3-L1-derived adipocytes ( a – f , h ) and MEF-derived adipocytes ( g ). All data are presented as mean±s.e.m. analysis of variance followed by Tukey–Kramer’s post hoc test; * P <0.05; ** P <0.005; NS, not significant. ( i ) Schematic diagram of the mechanism for GPR43-mediated suppression of fat accumulation. Novel GPR43 signalling events in adipocytes are shown in red. Full size image Next, we examined whether GPR43 directly suppresses insulin signalling. Acetate significantly promoted phosphorylation of PTEN (phosphatase and tensin homologue), a negative regulator of insulin/PI3K signalling [35] , and the effect was effectively blocked by treatment with Go6983 and PTX ( Fig. 5e ). In addition, acetate-mediated suppression of insulin-induced Akt phosphorylation was effectively blocked by treatment with bpV(pic), a PTEN inhibitor ( Fig. 5f ). PKC-dependent phosphorylation of liver kinase B1 (LKB1) is reported to promote PTEN phosphorylation [36] . Acetate significantly promoted phosphorylation of LKB1 with or without insulin, and the effect was effectively blocked by treatment with Go6983 and PTX ( Supplementary Fig. S4f ). On the other hand, acetate had no effect on insulin receptor substrate1, an insulin signalling adaptor protein [35] ) phosphorylation ( Supplementary Fig. S4g ). In addition, acetate significantly suppressed epidermal growth factor-induced Akt phosphorylation ( Supplementary Fig. S4h ). Moreover, treatment with acetate or PA significantly suppressed insulin-induced glucose uptake and LPL activation, and these inhibitory effects were abolished by treatment of PTX ( Fig. 5g ). Thus, acetate-mediated activation of GPR43 suppresses the bioactivity of insulin by suppression of Akt phosphorylation via G(i/o)βγ–PLC–PKC–PTEN ( Fig. 5i ). GPR43 promotes energy expenditure We finally assessed the effects on energy metabolism exerted by adipose GPR43. The plasma triglyceride content in HFD-fed Gpr43−/− mice was markedly low compared with wild-type mice, whereas that in aP2-Gpr43TG mice was markedly high ( Fig. 6a ). These differences were abolished under GF conditions or by treatment with antibiotics ( Supplementary Fig. S5a,b ). However, the plasma free-fatty acid ( Fig. 6b ), glucose ( Supplementary Fig. S5c ) and insulin ( Supplementary Fig. S5d ) levels were comparable between wild-type and Gpr43−/− mice fed an HFD and between wild-type and aP2-Gpr43TG mice. Hence, changes in systemic insulin sensitivity observed in Gpr43−/− and aP2-Gpr43TG mice are not due to abnormal secretion of insulin. These results suggested that lipids and glucose were not taken up into adipose tissues and were instead consumed by other tissues. As expected, the expression of energy expenditure-, glycolysis- and β-oxidation-related genes were increased, while the expression of gluconeogenesis-related genes were decreased in the muscles, but not the liver of aP2-Gpr43TG mice ( Fig. 6c ; Supplementary Fig. S5e ). To assess the energy expenditure and substrate utilization, we performed indirect calorimetry of wild-type and mutant mice. The Gpr43−/− mice showed decreased energy expenditure compared with wild-type mice fed an HFD ( Fig. 6d ), although both groups of mice showed similar locomotor activity ( Fig. 6e ). In contrast, aP2-Gpr43TG mice showed an increased energy expenditure compared with wild-type mice during all phases ( Fig. 6g ), although both groups of mice showed similar levels of locomotor activity during the light phase ( Fig. 6h ). Moreover, interestingly, although Gpr43−/− mice showed obesity and aP2-Gpr43TG mice showed leaness compared with wild-type mice fed an HFD, the respiratory exchange ratio (RER) was higher in Gpr43−/− and lower in aP2-Gpr43TG mice than in wild-type mice ( Fig. 6f ). The RER is reduced because of preferential utilization of fat during obesity [37] . Collectively, our results indicated that GPR43 activation promoted energy expenditure and permitted the preferential utilization of fat as a fuel through suppression of fat accumulation by inhibition of adipose tissue-specific insulin signalling. 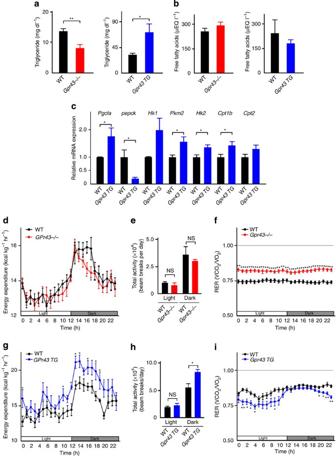Figure 6: GPR43 promotes energy expenditure by increasing the consumption of lipids. Biochemical analysis of plasma obtained fromGpr43−/−mice on an HFD as well asaP2-Gpr43TGmice: triglycerides (a,n=6–7); free fatty acids (b,n=5–9). (c) mRNA levels of genes involved in energy expenditure (Pgc1a), gluconeogenesis (Pepck), glycolysis (Hk1,Pkm2, andHk2) and β-oxidation (Cpt1bandCpt2) in the muscles ofaP2-Gpr43TGmice on an HFD (n=4). (d) Energy expenditure ofGpr43−/−mice on an HFD (n=7). (e) Total activity inGpr43−/−mice fed an HFD (n=5, 3). (f) RER ofGpr43−/−mice fed an HFD (n=7). (g) Energy expenditure ofaP2-Gpr43TGmice (n=7). (h) Total activity inaP2-Gpr43TGmice (n=5, 4). (i) RER ofaP2-Gpr43TGmice (n=7). All mice were analysed at 16 weeks of age. All data are presented as mean±s.e.m. Student’st-test; *P<0.05; **P<0.005; NS, not significant. Figure 6: GPR43 promotes energy expenditure by increasing the consumption of lipids. Biochemical analysis of plasma obtained from Gpr43−/− mice on an HFD as well as aP2-Gpr43TG mice: triglycerides ( a , n =6–7); free fatty acids ( b , n =5–9). ( c ) mRNA levels of genes involved in energy expenditure ( Pgc1 a), gluconeogenesis ( Pepck ), glycolysis ( Hk1 , Pkm2 , and Hk2 ) and β-oxidation ( Cpt1b and Cpt2 ) in the muscles of aP2-Gpr43TG mice on an HFD ( n =4). ( d ) Energy expenditure of Gpr43−/− mice on an HFD ( n =7). ( e ) Total activity in Gpr43−/− mice fed an HFD ( n =5, 3). ( f ) RER of Gpr43−/− mice fed an HFD ( n =7). ( g ) Energy expenditure of aP2-Gpr43TG mice ( n =7). ( h ) Total activity in aP2-Gpr43TG mice ( n =5, 4). ( i ) RER of aP2-Gpr43TG mice ( n =7). All mice were analysed at 16 weeks of age. All data are presented as mean±s.e.m. Student’s t -test; * P <0.05; ** P <0.005; NS, not significant. Full size image SCFAs, including acetate, act as ligands for GPR43 and are produced by gut microbiota [12] . Under HFD-fed conditions, faecal SCFA and plasma acetate contents in HFD-fed mice significantly decreased compared with those in NC-fed mice ( Supplementary Fig. S2a,b ). This is presumably due the replacement of carbohydrate with fat in the HFD, which reduced SCFA production by gut microbiota ( Supplementary Table S1 ). However, Gpr43 expression was markedly higher (approximately twice) in the WAT of HFD-fed mice as compared with NC-fed mice ( Fig. 1e ). This indicates that although there was a decrease of endogenous SCFA ligands, the increase of GPR43 expression in adipose tissue contributed to the dramatic phenotype in Gpr43−/− mice, which is further exacerbated by the HFD-induced metabolic phenotype. GPR43 promotes leptin secretion and adipogenesis, and inhibits lipolysis in vitro [19] , [22] , [23] , [24] . However, our studies, using Gpr43−/− mice and aP2-Gpr43TG mice, showed that adipogenesis was comparable in wild-type, Gpr43−/− and aP2-Gpr43TG mice at the P1. Moreover, the plasma leptin levels were comparable in wild-type and Gpr43−/− mice. In contrast, the plasma leptin level in aP2-Gpr43TG mice was lower than in wild-type mice at the adult stage. These results suggested that the in vitro experiments did not correctly reflect the physiological conditions in vivo . Furthermore, the in vivo experiments showed that the inhibition of lipolysis by GPR43 activation decreased the plasma free-fatty acid level, and the response abolished in Gpr43−/− mice [23] . These responses may be explained by the suppression of fat intake in the WAT via inhibition of insulin signalling but not lipolysis. Hence, by integrating the function of GPR43 in the WAT, including inhibition of LPL activity, glucose uptake and lipid uptake, our current study clarified that GPR43 activation leads to the suppression of insulin signalling and thereby prevents energy accumulation. Recently, some controversy appeared concerning the role of GPR43 in the regulation of the energy balance in vivo . One study showed that activation of GPR43 enhanced insulin sensitivity by promoting GLP-1 secretion in the gut [26] . On the other hand, GPR43 deficiency also improved insulin sensitivity and protected against HFD-induced obesity and dyslipideamia via increased energy expenditure at older ages (7–8 months of age) but an otherwise unclear mechanism [25] . Our results support the former study as our GPR43-deficient mice exhibited obesity and impaired systemic insulin sensitivity, whereas our aP2-Gpr43TG mice exhibited leanness and enhanced systemic insulin sensitivity. In the adipose tissue, in particular, aP2-Gpr43TG reflected the phenotype of Gpr43−/− mice, suggesting that lipid metabolism and fat accumulation in the adipose tissue are modulated by adipose-expressed GPR43. We also confirmed the decrease and increase in systemic insulin sensitivity by insulin clamp test in HFD-fed Gpr43−/− mice ( Fig. 2i ) and aP2-Gpr43TG mice ( Fig. 3q ), respectively. Moreover, other group reported that resistant starch supplementation leads to an increase of SCFAs, and systemic and muscle insulin sensitivity, although systemic FFA concentrations were not altered and LPL activity was decreased [38] . Hence, this report also supports Tolhurst et al. [26] and our results. In addition, the differences between the three knockout models, including ours, may reflect differences in the genetic backgrounds or the variation in the gut microbiota composition under different environments. Hence, we further examined whether the difference of genetic backgrounds of each mice (Bjursell et al . : C57BL/6 mice, our study: 129/SvEv mice) and the rearing environments influence to the difference of phenotype. At first, we backcrossed 129 background Gpr43−/− mice into C57B/6J (more than 10 times). The difference of body weight between B6 backcrossed Gpr43−/− and wild-type mice were attenuated compared with that of the 129 background. Nevertheless, B6 backcrossed Gpr43−/− mice also exhibited tendency of increase of body weight ( Supplementary Fig. S6c ). Next, we examined SCFAs production in mice under different environment, namely, mice housed in shoebox-style cages (CONV conditions), and mice housed in cages in an isolation rack ventilated with sterilized air from the backside of each rack (specific pathogen-free conditions; SPF), because microbiota community under CONV condition remarkably differ from that under SPF condition [39] . Interestingly, faecal SCFAs contents and plasma acetate under CONV condition were significantly higher than that under SPF condition ( Supplementary Fig. S6d,e ), presumably for change of gut microbiota composition by different environment. Hence, GPR43 may be activated much more under our experimental environments, because all in vivo experiments in this study performed under CONV condition. Moreover, although weight gain of B6 mice had no difference between CONV and SPF condition, weight gain of 129 mice under CONV condition were significantly suppressed compared with that under the SPF condition ( Supplementary Fig. 6f ). These results indicate that intensity of the phenotype maybe influenced by the difference of environment and strain. Although GPR43 is a Gi/o- and Gq-dual-coupled GPCR [18] , [19] , recent studies have shown that all GPR43 functions are mediated by Gi/o; no functions involving Gq have been reported for GPR43 in adipose tissues [24] , [25] . Only in the intestine, GPR43 has been reported to promote GLP-1 secretion in L cells via the Gq protein [27] . Our study also showed that GPR43 signalling in WAT is mediated by Gi/o but not Gq. Hence, GPR43 may interact with only Gi/o in the WAT. Moreover, our results showed that GPR43 suppresses Akt phosphorylation by activating PTEN via G(i/o)βγ–PLC–PKC signalling and thereby inhibits fat accumulation in WAT. We also showed that GPR43 was abundantly expressed in the WAT but was barely expressed in the BAT, muscles and liver, where they acted as an insulin effectors ( Fig. 1a ). Although GPR43 suppress insulin signalling in WAT ( Fig. 4 ), ITT and glucose clamp test revealed that systemic insulin sensitivity was impaired in Gpr43−/− mice and enhanced in aP2-Gpr43TG mice ( Figs 2g , i and ). Glucose clamp test further suggested that adipose GPR43 improves insulin sensitivity in other tissues such as liver and muscle. HGP suppression ( Figs 2i and 3q ) demonstrated the hepatic insulin resistance, and the decreased Rd ( Figs 2i and 3q ) strongly suggested insulin resistance in muscle, because 70–80% of total body insulin-stimulated glucose disposal is accounted for by skeletal muscle glucose uptake [40] . Moreover, energy expenditure- and glycolysis-related genes in muscle of aP2-Gpr43TG mice increased ( Fig. 6c ). Consequently, GPR43 enhances energy utilization in other tissues except for adipose tissues. In addition, adipose tissue-selective knockout of the insulin receptor in mice protects against obesity and obesity-related glucose intolerance [41] . Hence, this report also supports our results that suppression of adipose insulin signalling by GPR43 activation leads to prevention of obesity and improves systemic insulin sensitivity. SCFAs are considered to be important energy sources for the host [42] , [43] . On the other hand, our present study revealed that SCFAs also act as signalling molecules for maintaining energy balance. Feeding increased the plasma glucose and lipid levels, and excess fatty acids and glucose were stored efficiently as fat. However, fat accumulation by excess feeding leads to obesity and induces several metabolic disorders. Our results showed that the plasma SCFA levels increases following a rise in plasma glucose level during feeding. Hence, GPR43 may function as an energy sensor to promote the utilization of excess energy in other tissue rather than storing excess energy as fat in the adipose tissue, thereby maintains metabolic homoeostasis. Moreover, GF conditions and treatment with antibiotics completely abolished the metabolic dysfunction-related phenotype in GPR43-mutant mice, indicating that the gut microbiota is the most important supplier of GPR43 agonists and that the functions of GPR43 are closely linked to the gut microbiota. In this study, we showed that SCFAs activate GPR43 to regulate the energy uptake in WAT, which leads to the regulation of energy expenditure in other tissues, including liver and muscle. We also reported that GPR41, another SCFA receptor, regulates body energy expenditure by activating sympathetic nervous system at the level of ganglion [14] . These findings indicate that SCFAs produced by gut microbiota, through activation of GPR41 and GPR43, have important roles in recognition of postprandial nutrient excess and orchestration of energy expenditure to maintain energy homoeostasis ( Fig. 7 ). In addition, the results obtained in our GPR43-overexpression mouse model indicate the possibility that overstimulation of GPR43 could be a strategy for therapy of metabolic disorders, including obesity and diabetes mellitus. 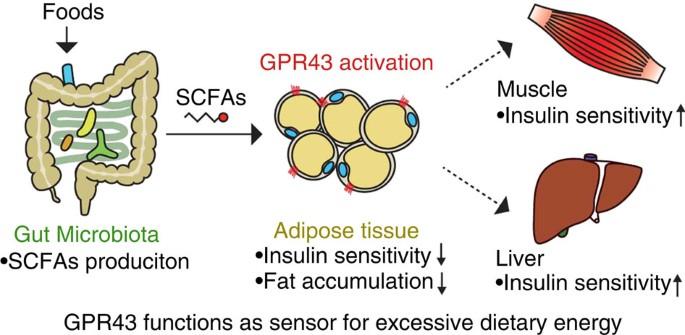Figure 7: Schematic model of suppression of fat accumulation via GPR43. After feeding, SCFAs, produced by microbial fermentation in the gut, activate GPR43 in adipose tissues. SCFA-mediated GPR43 activation suppresses insulin-mediated fat accumulation and thereby regulates the energy balance by suppressing accumulation of excess energy and promoting fat consumption. Figure 7: Schematic model of suppression of fat accumulation via GPR43. After feeding, SCFAs, produced by microbial fermentation in the gut, activate GPR43 in adipose tissues. SCFA-mediated GPR43 activation suppresses insulin-mediated fat accumulation and thereby regulates the energy balance by suppressing accumulation of excess energy and promoting fat consumption. Full size image Animals Mice were housed under a 12-h light–dark cycle and given NC (MF, Oriental Yeast Co.). For HFD studies, 4-week-old male mice were placed on a 58Y1 diet (PMI Nutrition International) for 12 weeks. The composition of the diets is given in Supplementary Table S1 . All experimental procedures involving mice were performed according to protocols approved by the relevant Animal Ethics Committees. Gpr43−/− mice from a 129/Sv background and aP2-Gpr43TG mice (Acc. No. CDB0480T, http://www.cdb.riken.jp/arg/TG%20mutant%20mice%20list.html ) from a C57BL/6 background were generated. GF mice were obtained from CLEA Japan Inc. (Tokyo, Japan) and bred in the Central Institute For Experimental Animals (Kanagawa, Japan). Surveillance for bacterial contamination was performed by periodic bacteriological examination of faeces throughout the experiments. For microbiota transplantation, faecal contents were pooled from four age- and gender-matched wild-type CONV mice. Faecal extracts were suspended in PBS and then administered. For antibiotic treatment, 4-week-old mice were treated with ampicillin (1.0 mg ml −1 ) and neomycin (0.5 mg ml −1 ) in drinking water for 12 weeks [28] . For acetate administration, 4-week-old mice were treated with sodium acetate (150 mM) in drinking water for 12 weeks [20] . In situ hybridization Mouse embryos were frozen in optimum cutting temperature compound (Sakura Finetech), and 18-μm sections were cut using a cryostat and stored at −80 °C until hybridization. Mouse and human antisense Gpr43 RNA probes were transcribed using T7 RNA polymerase with uridine 5′-α-[ 35 S]-thio-triphosphate (Perkin Elmer). Sections were examined as described [14] , and counterstained with haematoxylin–eosin and oil red O (Sigma) for liquid deposition. RNA isolation and real-time quantitative RT-PCR Total RNA was extracted using the RNeasy Mini Kit (Qiagen) and ISOGEN (WAKO). Complementary DNAs were transcribed using RNAs as templates with Moloney murine leukaemia virus reverse transcriptase (Invitrogen). cDNAs were amplified by PCR with Taq DNA polymerase (TaKaRa) using the primers listed in Supplementary Table S2 . Real-time quantitative RT-PCR (qRT-PCR) analyses were performed using DNA Engine Opticon-2 (MJ Research) as described [14] . The expression was quantified in duplicate. Quantification of faecal microbiota by qRT-PCR DNA was extracted from frozen extruded faecal contents using the QIAamp DNA Stool Mini Kit (Qiagen) under modified manufacturer instructions. Briefly, frozen faeces was heated at 65 °C for overnight. Approximately 220 mg of dry stool samples were homogenized and heated at 95 °C for 5 min. After incubation with an Inhibit Ex Tablet (Qiagen), the lysates were treated with proteinase K and buffer AL at 70 °C for 10 min. DNA was purified using a column provided in the kit [44] . DNA was then quantified as described [45] , [46] using the primers listed in Supplementary Table S3 . Histology Adipose tissues were fixed in 10% neutral-buffered formalin, embedded in paraffin and sectioned (5 μm). Haematoxylin–eosin staining was performed using the standard techniques. To measure the diameter of the adipocytes, the diameters of 100 cells from five sections from each group were measured using NIH IMAGE J. More than 10 fields were examined, and the results were expressed as the average. Liver tissues were embedded, frozen and sectioned (16 μm). The sections were stained with oil red O (Sigma) for lipid deposition as described [47] . Immunohistochemstry was performed by using antibodies against F4/80 (Abcam; rat, 1:1,000) and Caveolin1 (BD Biosciences; mouse, 1:200) as described [48] . Triglyceride content assay The liver was homogenized with acetic acid (0.5 M)/methanol/chloroform at relative proportions of 1/2.5/1.25 (v/v/v). The mixture was shaken, and 1.25 volumes of chloroform were added. The mixture was shaken overnight and 1.25 volumes of 0.5 M acetic acid was added. After centrifugation at 1,500 g for 10 min, the organic layer was collected, dried and resuspended in 100% isopropyl alcohol. Measurements were conducted using the Triglyceride E-test (Wako, Japan) as described [47] . GTT and ITTs For GTT, 24-h-fasted mice were given 1.5 mg of glucose per gram of body weight intraperitoneally (i.p.). For ITT, 3-h-fasted mice were given human insulin (0.75 mU g −1 , i.p., Sigma). The plasma glucose concentration was monitored before injection and at 15, 30, 60, 90 and 120 min after injection. Hyperinsulinaemic euglycaemic clamp Hyperinsulinaemic euglycaemic clamp studies were performed after 4–6 days of recovering from cannulization as described previously with minor modification [49] . During clamp studies, human insulin was infused at 3 mU kg −1 min −1 into mice, with variable amounts of 40% glucose solution to maintain a blood glucose level of 90–120 mg dl −1 . The blood glucose was measured every 10 min. GIR and endogenous glucose production were measured between 90 and 120 min after the initiation of insulin infusion. Assay of biochemical responses to insulin stimulation Insulin (0.15 U kg −1 , Sigma) was injected i.p. After 5 min, liver, skeletal muscle or WAT were dissected and immediately frozen in liquid nitrogen. Immunoblot analysis was performed as described [47] . Adipocyte culture MEFs and 3T3-L1 pre-adipocytes (ATCC) were cultured at 37 °C in α-MEM (for MEFs) or Dulbecco’s modified Eagle’s medium (DMEM, for 3T3-L1) containing 1% penicillin–streptomycin solution (Gibco) with 10% fetal bovine serum (FBS). Two days after confluence, the medium was replaced with α-MEM or DMEM containing 10% FBS and inducers (0.25 μM dexamethasone, 10 μg ml −1 insulin, and 0.5 mM 3-isobutyl-1-methylxanthine) as well as pioglitazone (10 μM) for 2 days. The medium was then changed to DMEM supplemented with 10% FBS, 10 μg ml −1 insulin and 10 μM pioglitazone, and then incubated for 2 days. After 5 days, the differentiated adipocytes were used for experiments [50] . Glucose uptake assay The epididymal fat pads were minced and washed with KRBH (Krebs-Ringer bicarbonate solution buffered with 30 mM HEPES, pH 7.4, containing 2.5 mM glucose and 1% (w/v) fatty-acid-free bovine serum albumin (Sigma), and were incubated with collagenase type 2 (1 mg ml −1 , Sigma) at 37 °C. After 15 min, the content was filtered and washed with KRBH without glucose. The floating cells or MEF-derived adipocytes were incubated with KRBH without glucose for 30 min or 3 h, respectively, with or without acetate (10 mM). After incubation with insulin (3 μg ml −1 ) for 20 min at 37 °C, 0.1 mM 2-deoxyglucose (Sigma) and 1 μCi [ 3 H]-2-deoxyglucose (Moravek Biochemicals) were added, and incubated for 10 min at 37 °C. The adipocytes were washed three times with ice-cold KRBH with 2.5 mM glucose, and the level of radioactivity was counted [51] . Fatty acid uptake assay MEF-derived adipocytes were plated into 96-well black-well, clear-bottom plates. Cells were serum deprived for 1 h, with or without acetate (10 mM), before treatment with insulin (3 μg ml −1 ) for 30 min. QBT Fatty Acid Uptake solution (Molecular Probes) was then added. After 1 h, the fluorescence intensity was measured using a Wallac 1420 ARVOsx (Perkin Elmer). Biochemical analyses The plasma glucose concentrations was measured using a One Touch Ultra (LifeScan). Measurements of the plasma FFA and triglyceride concentration was performed in SRL Inc. The plasma acetate concentration was measured using F-kit acetate (Boehringer Mannheim). Measurements of faecal SCFAs by ion chromatography (IC) were entrusted to the Kyoto Institute of Nutrition and Pathology Inc. LPL activity assay Tissues were homogenized in 0.1 M sodium phosphate, pH 7.4, and centrifuged at 10,000 g for 20 min at 4 °C. The LPL activity was measured by using an LPL assay kit (Roar Biomedicals). For differentiated 3T3-L1 cells, cells were pretreated with PTX (1 μg ml −1 ) in complete medium for 2 h. Adenosine A1 receptor, a Gi/o-coupled GPCR, is constitutively activated by endogenous adenosine [32] . Hence, the cells were pretreated with 1% BSA (fatty acids free) and adenosine deaminase (1 U ml −1 ) for 2 h to suppress increase of LPL activity by PTX-induced suppression of this receptor. Next, the cells were serum deprived for 2 h with or without acetate (10 mM), and PTX (1 μg ml −1 ) before treatment with insulin (3 μg ml −1 ) for 30 min, followed by treatment with heparin (100 U/ml −1 , Ajinomoto) for 10 min. The culture medium was then removed and assayed. Indirect calorimetry The oxygen consumption (VO 2 ) and RER were determined with an O 2 /CO 2 metabolic measuring system (Model MK-5000, Muromachi Kikai) at 24 °C as described [14] . VO 2 was expressed as the volume of O 2 consumed per kilogram of lean body mass weight per minute. The energy expenditure was calculated as the product of the calorific value of oxygen (3.815+1.232 × RER) and VO 2 [47] . The locomotor activity was measured by using an infrared-ray passive sensor system (Supermex, Muromachi Kikai Co.). Knockdown by siRNA Adipocytes were transfected with 40 nM siRNA shown in Supplementary Table S4 (Stealth Select RNAi, Invitrogen) using the Lipofectamine RNAiMAX transfection reagent (Invitrogen) as described [14] . Western blotting Cells were lysed in TNE buffer. Tissues were homogenized in 0.1 M sodium phosphate buffer, pH 7.4, and centrifuged at 10,000 g for 20 min at 4 °C. The supernatants were analysed by western blotting using antibodies targeting Akt, phosphorylated Akt (Ser473), ERK1/2, phosphorylated ERK1/2, aP2, PPARg, phosphorylated PTEN (Ser380/Thr382/383), PTEN, phosphorylated LKB1 (Ser428), LKB1 (Cell signaling; rabbit, 1:1,000), Gq (Santa Cruz; rabbit, 1:200) and β-actin (Sigma; mouse, 1:1,000). The immunoreactive bands were visualized as previously described [14] . Statistical analyses Values are presented as the mean±s.e.m. Differences between groups were examined for statistical significance using Student’s t -test (two groups) or analysis of variance (≥3 groups). P -values<0.05 were considered statistically significant. How to cite this article: Kimura, I. et al. The gut microbiota suppresses insulin-mediated fat accumulation via the short-chain fatty acid receptor GPR43. Nat. Commun. 4:1829 doi: 10.1038/ncomms2852 (2013).